Spin-valley lifetimes in a silicon quantum dot with tunable valley splitting Although silicon is a promising material for quantum computation, the degeneracy of the conduction band minima (valleys) must be lifted with a splitting sufficient to ensure the formation of well-defined and long-lived spin qubits. Here we demonstrate that valley separation can be accurately tuned via electrostatic gate control in a metal–oxide–semiconductor quantum dot, providing splittings spanning 0.3–0.8 meV. The splitting varies linearly with applied electric field, with a ratio in agreement with atomistic tight-binding predictions. We demonstrate single-shot spin read-out and measure the spin relaxation for different valley configurations and dot occupancies, finding one-electron lifetimes exceeding 2 s. Spin relaxation occurs via phonon emission due to spin–orbit coupling between the valley states, a process not previously anticipated for silicon quantum dots. An analytical theory describes the magnetic field dependence of the relaxation rate, including the presence of a dramatic rate enhancement (or hot-spot) when Zeeman and valley splittings coincide. Silicon is at the heart of all modern microelectronics. Its properties have allowed the semiconductor industry to follow Moore’s law for nearly half a century, delivering nowadays billions of nanometre-scale transistors per chip. Remarkably, silicon is also an ideal material to manipulate quantum information encoded in individual electron spins [1] , [2] , [3] . This is a consequence of the weak spin–orbit coupling and the existence of an abundant spin-zero isotope, which can be further enriched to obtain a ‘semiconductor vacuum’ in which an electron spin can preserve a coherent quantum superposition state for exceptionally long times [4] . In order to define a robust spin-1/2 qubit Hilbert space, it is necessary that the energy scale of the two-level system is well separated from higher excitations. In this respect, a major challenge for the use of silicon is represented by the multi-valley nature of its conduction band. In a bulk silicon crystal the conduction band minima are six-fold degenerate, but in a two-dimensional electron gas (2DEG), the degeneracy is broken [5] into a two-fold degenerate ground state (Γ valleys) and a four-fold degenerate excited state (Δ valleys), owing to vertical confinement of electrons with different effective mass along the longitudinal and transverse directions, respectively. Furthermore, the Γ valley degeneracy is generally lifted by a sharp perpendicular potential [6] , [7] , [8] , [9] and the relevant energy separation is termed valley splitting (VS). The VS depends on physics at the atomic scale [10] , [11] , [12] (for example, roughness, alloy and interface disorder), and so it is not surprising that experiments have revealed a large variability of splittings among devices, ranging from hundreds of μeV [5] , [13] , [14] , [15] up to tens of meV in exceptional cases [16] . At present, the lack of a reliable experimental strategy to achieve control over the VS is driving an intense research effort for the development of devices that can assure robust electron spin qubits by minimizing multi-valley detrimental effects [17] , [18] , or even exploit the valley degree of freedom [19] , [20] for new types of qubits. Another crucial parameter to assess the suitability of a physical system to encode spin-based qubits is the relaxation time of spin excited states ( T 1 ). Spin lifetimes have been measured for gate-defined Si quantum dots (QDs) [21] , Si/SiGe QDs [22] , [23] and donors in Si (ref. 24 ), reporting values that span from a few milliseconds to a few seconds. Furthermore, the dependence of the spin relaxation rate ( ) on an externally applied magnetic field ( B ) has been investigated. Different mechanisms apply to donors and QDs, accounting for the observed B 5 and B 7 dependencies [25] , respectively. In principle, ( B ) depends on the valley configuration and the details of the excited states above the spin ground state. However, until now, no experimental observation of the effects of a variable VS on the relaxation rate has been reported. Here, we demonstrate for the first time that the VS in a silicon QD can be finely tuned by direct control of an electrostatic gate potential. We find that the dependence of the VS on vertical electric field at the Si/SiO 2 interface is strikingly linear, and show that its tunability is in excellent agreement with atomistic tight-binding predictions. We demonstrate accurate control of the VS over a range of about 500 μeV and use it to explore the physics of spin relaxation for different QD occupancies ( N =1, 2, 3). We probe both the regime where the VS is much larger than the Zeeman splitting at all magnetic fields and that where the valley and spin splittings are comparable. We observe a dramatic enhancement of the spin decay rate (relaxation hot-spot) when spin and valley splittings coincide. To our knowledge, such hot-spots have been predicted for relaxation involving orbital states [26] , [27] (not valley states), but these are yet to be observed. We develop an analytic theory that explains the B -field dependence of the relaxation rates and the details of the relaxation hot-spot in terms of admixing of spin-valley states. This mechanism is seen to be significantly more prominent than the conventional spin–orbit hybridization [28] . QD addition spectrum Our device is fabricated using a multi-level gated metal–oxide–semiconductor (MOS) technology [29] , and its architecture is depicted in Fig. 1a–d . A quantum dot is formed under gate P by applying a positive bias voltage to induce an electron accumulation layer. Strong planar confinement for the dot’s potential well is achieved by negatively biasing gates B, C1 and C2. A 2DEG reservoir is also induced by positively biasing gates R1 and R2, and the QD occupancy can be modified by inducing electrons to tunnel between this reservoir and the dot. The remaining gates, namely, SB1, SB2 and ST, are employed to define a single-electron transistor (SET), capacitively coupled to the QD and used as a read-out device. The high flexibility of our design would allow us to use the same device also as a (single-lead) double-dot structure by rearranging the gate bias (for example, dots can be formed under gates B and C2). However, in this work, we only present results relevant to the single-dot configuration. 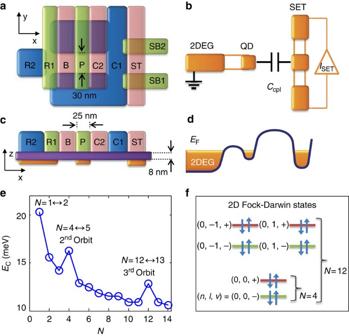Figure 1: Device architecture and addition energy spectrum. (a) Schematic (top view) of the device’s gate layout. Different colours represent different layers within the gate stack. (b) Schematic diagram of the single-lead QD (left) and SET detector (right). Regions where an electron layer is formed are coloured in orange. The read-out signal (ISET) is sensitive to the QD charge state due to the QD/SET capacitive coupling (Ccpl). (c) Device cross-sectional schematic. An electron layer is formed underneath the positively biased gates: R1 and R2 define the QD reservoir; P controls the QD population, and ST the sensor’s island. The SiO2layer (in purple) thickness and plunger gate width are indicated. (d) Energy diagram showing qualitatively the conduction band profile in the device. Electrons accumulate wherever the gate bias lowers the conduction band below the Fermi level,EF. (e) Charging energy as a function of electron number. Spikes corresponding to complete 2D shell filling are observed. (f) Schematic of electron filling for two-valley 2D Fock–Darwin states. Each state can hold two electrons of antiparallel spin and is identified by a pair of quantum numbers (n,l) and its valley occupancy (v). Figure 1: Device architecture and addition energy spectrum. ( a ) Schematic (top view) of the device’s gate layout. Different colours represent different layers within the gate stack. ( b ) Schematic diagram of the single-lead QD (left) and SET detector (right). Regions where an electron layer is formed are coloured in orange. The read-out signal ( I SET ) is sensitive to the QD charge state due to the QD/SET capacitive coupling ( C cpl ). ( c ) Device cross-sectional schematic. An electron layer is formed underneath the positively biased gates: R1 and R2 define the QD reservoir; P controls the QD population, and ST the sensor’s island. The SiO 2 layer (in purple) thickness and plunger gate width are indicated. ( d ) Energy diagram showing qualitatively the conduction band profile in the device. Electrons accumulate wherever the gate bias lowers the conduction band below the Fermi level, E F . ( e ) Charging energy as a function of electron number. Spikes corresponding to complete 2D shell filling are observed. ( f ) Schematic of electron filling for two-valley 2D Fock–Darwin states. Each state can hold two electrons of antiparallel spin and is identified by a pair of quantum numbers ( n , l ) and its valley occupancy ( v ). Full size image In order to characterize the addition spectrum of the QD, we make use of a technique previously developed for GaAs-based systems, which combines charge detection and gate pulsing [30] . There is no direct transport through the single-lead QD and, therefore, addition/removal of charge is only detected via modifications in the SET current. In particular, charge transitions are detected as current peaks in the SET signal whenever the QD energy eigenstates come into resonance with the reservoir’s Fermi level. Note that the SET–QD coupling is merely capacitive (via C cpl ) and electrons do not tunnel between them. In order to maximize charge sensitivity in the detector, we employ dynamic voltage compensation [31] on different gates, which makes our read-out signal virtually unaffected by slow charge drifts and random charge rearrangements. A comprehensive discussion of the charge stability measurements can be found in Supplementary Note 1 . Figure 1e illustrates the addition energy spectrum for the first 14 electron additions to the QD. There is very little variation of charging energy ( E C ) for high occupancies ( E C ≈ 11 meV for N >9). However, by decreasing the electron number, the charging energy steadily increases, as expected when the dot size is significantly affected by the electron number. This evidently indicates that the few-electron regime has been achieved. Most interestingly, the energy spectrum shows peaks for the addition of the fifth and thirteenth electrons. The extra addition energy needed for those transitions can be attributed to complete filling of the first and second orbital shells. As illustrated in Fig. 1f , this is consistent with the energy spectrum of two-valley 2D Fock–Darwin states [32] , where the first and second orbital shells hold four and eight electrons, respectively. This confirms that we can probe the occupancy until the last electron. To our knowledge, such a clear manifestation of two-dimensional shell structure has been observed before only in InGaAs dots [33] and in Si/SiGe dots [34] . Spin-valley lifetimes In order to measure the spin state of individual electrons in the QD, we use an energy-selective read-out technique [35] . The read-out protocol consists of three phases clocked by a three-level pulsed voltage applied to gate P, which directly controls the dot’s electrochemical potential (see Fig. 2a ). First, an electron of unknown spin is loaded into the dot, causing a sudden decrease in the sensor current. Next, the potential of the dot is lifted so that the Fermi level of the reservoir lies between the spin-up and spin-down states of the dot, meaning that a spin-up electron can tunnel off the dot while a spin-down electron is blocked. This is the read phase, during which the presence of a spin-up state would be signalled by a current transient (spin-up tunnels out and then spin-down tunnels in) whereas a spin-down electron would lead to no current modification. Finally, the dot’s potential is further lifted to allow the electron to tunnel off, regardless of its spin orientation. In Fig. 2b , single-shot traces for both spin-up (in blue) and spin-down (in green) detection are plotted. The longer the system is held in the load phase before performing a read operation, the more likely it is for the spin-up excited state to decay to the spin-down ground state. Thus, by varying the length of the load phase and monitoring the probability of detecting a spin-up electron, we can determine [35] , [24] the spin lifetime, T 1 . In our experiments the B field is directed along the [110] crystallographic axis. A comprehensive discussion of both the spin-up fraction measurements and the fitting procedure to evaluate T 1 is included in the Supplementary Note 2 . As shown in Fig. 2d , we observe a wide range of spin lifetimes as a function of magnetic field, with lifetimes as long as 2.6 s at the lowest fields studied, B =1.25 T. These are some of the longest lifetimes observed to date in silicon quantum dots [25] . 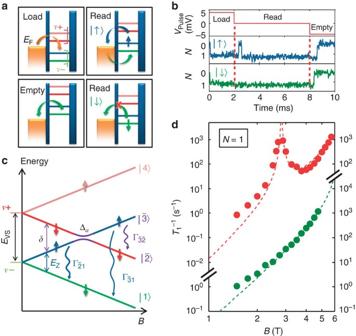Figure 2: Spin read-out and relaxation rates for single-electron occupancy. (a) Schematic diagram showing the effect of the three-level pulse sequence on the electro-chemical potential of the dot. Energy levels in the QD are Zeeman split according to spin polarization and valley degeneracy is lifted. For clarity, only lower valley states are shown to be loaded/unloaded. (b) Pulsing sequence (top) for the single-shot spin read-out and normalised SET signal for spin-up (middle) and spin-down (bottom). (c) Energy diagram of the one-electron spin-valley states as a function ofBfield. Maximum mixing of spin and valley degrees of freedom occurs at the anticrossing point where Zeeman and valley splittings coincide. Relevant relaxation processes are sketched. (d) Relaxation rates as a function of magnetic field for different valley splittings. Data points forEVS=0.75 meV,EVS=0.33 meV are shown as green and red circles, respectively. Dashed lines are the calculated relaxation rates fitted withr=1.7 nm (green),r=1.1 nm (red). Figure 2: Spin read-out and relaxation rates for single-electron occupancy. ( a ) Schematic diagram showing the effect of the three-level pulse sequence on the electro-chemical potential of the dot. Energy levels in the QD are Zeeman split according to spin polarization and valley degeneracy is lifted. For clarity, only lower valley states are shown to be loaded/unloaded. ( b ) Pulsing sequence (top) for the single-shot spin read-out and normalised SET signal for spin-up (middle) and spin-down (bottom). ( c ) Energy diagram of the one-electron spin-valley states as a function of B field. Maximum mixing of spin and valley degrees of freedom occurs at the anticrossing point where Zeeman and valley splittings coincide. Relevant relaxation processes are sketched. ( d ) Relaxation rates as a function of magnetic field for different valley splittings. Data points for E VS =0.75 meV, E VS =0.33 meV are shown as green and red circles, respectively. Dashed lines are the calculated relaxation rates fitted with r =1.7 nm (green), r =1.1 nm (red). Full size image A key focus of our experiment was to electrostatically tune the valley energy separation and measure relaxation rates in different valley configurations and QD electron occupancies. As we show below, our data definitively indicate that excited valley states have a critical role in the spin relaxation processes. We develop a theory to explain how changes in the VS affect the spin-valley state mixing and leads to the observed relaxation times. As we detail in the following section, we have attained accurate gate control of the VS, allowing us to tune it over a range of hundreds of μeV. This permits us to conduct experiments in regimes where the VS ( E VS ) is either larger or smaller than the Zeeman spin splitting ( E Z ), depending on the magnitude of the magnetic field (see Fig. 2c ). Figure 2d presents measurements of spin relaxation rates as a function of magnetic field for two VS values at a fixed dot population of N =1. We start by examining a configuration where the valley separation is larger than the spin splitting at all fields (green data set). In other words, we operate in a regime for which where g is the electron gyromagnetic ratio, μ B is the Bohr magneton and B is the applied in-plane magnetic field. For E VS =0.75 meV (green data in Fig. 2d ), we observe a monotonic increase in the rate with respect to B that becomes increasingly fast as E Z approaches E VS . In our experimental conditions ( B field parallel to [110]), the B 5 dependences for known bulk-like mechanisms in silicon [36] , [37] should not apply, while predicted [23] , [25] , [27] , [38] rates B 7 do not explain the experimental data. By decreasing the valley separation to E VS =0.33 meV, we can achieve the condition where the Zeeman splitting matches or exceeds the VS. The red data in Fig. 2d illustrate the situation where inequality (1) only holds for B <2.8 T. When E Z = E VS (that is, for B =2.8 T), a spike in the relaxation rate occurs. Relaxation hot-spots have been previously predicted to occur for spin relaxation involving orbital states in single and coupled QDs [26] , [27] , [39] , [40] . To our knowledge, this is the first experimental observation of such a phenomenon. In order to understand the relaxation mechanisms, we have developed a model that takes into account the perturbations in pure spin states due to spin–orbit coupling (SOC), yielding eigenstates that are admixtures of spin and valley states. The four lowest spin-valley states (see Fig. 2c ) are defined as , , , . These states are considered to be only very weakly affected by higher excitations, such as orbital levels that are at least 8 meV above the ground state in our device [41] . In Supplementary Note 3 we detail how mixing to a 2 p -like orbital state leads to a B 7 dependence in and is, therefore, important mainly for high B fields (above the anticrossing point). At lower fields, the prominent mechanism is the spin-valley admixing, which we now discuss in detail. The relaxation between pure spin states is forbidden because the electron–phonon interaction does not involve spin flipping. However, in the presence of interface disorder, SOC can mix states that contain both the valley and spin degrees of freedom, thus permitting phonon-induced relaxation. Indeed, in the non-ideal case of QDs with a disordered interface, roughness can perturb the envelope function of both valleys (otherwise identical for ideal interfaces) and allows one to assume non-zero dipole matrix elements connecting the valley states (see Supplementary Note 3 ), such as , , (for ideal interfaces these are non-zero only due to a strongly suppressed Umklapp process). By means of perturbation theory, we define renormalized excited states and that can relax to the ground state , as they have an admixture of the state of the same spin projection (see Fig. 2c ). The details of the SOC Hamiltonian, H SO , and perturbation matrix are reported in Supplementary Note 3 . The leading-order wavefunctions are given by: where , , and is an expression involving the detuning from the anticrossing point, δ ≡ E VS − E Z , and the energy splitting at the anticrossing: where β D ( α R ) is the Dresselhaus (Rashba) SOC parameter, ħ is the reduced Planck’s constant and m t =0.198 m e is the transverse effective electron mass. By evaluating the relaxation rate via the electron–phonon deformation potentials (proportional to the deformation potential constants, ), we obtain the rate below the anticrossing as: where the pure-valley relaxation rates are (for longitudinal and transverse phonons): where ρ is the silicon mass density, v σ is the speed of sound in silicon, , are the angular integrals, and Δ E v′v and r are the energy difference and the dipole matrix element relevant to the transition, respectively (see also Supplementary Note 3 ). The experimental condition for which the hot-spot occurs (that is, E VS = E Z ) is modelled as an anticrossing point for the mixed states and . At that point, spin relaxation is maximized and approaches the valley relaxation rate, as δ →0 in equation (5). Above the anticrossing (that is, E VS < E Z ), the relevant relaxation transitions are and (the subsequent decay is in the form of a fast inter-valley transition, and is therefore neglected). The analytical formulations of these contributions read: The dashed lines in Fig. 2d show the calculated relaxation rates relevant to the two experimental values of E VS discussed, also including B 7 contribution from SOC mixing with the higher orbital state (see Supplementary Note 3 ). We use dipole matrix elements as a single free parameter by assuming . A least-square fit to the experimental data is performed by fixing the SOC strength to ( β D − α R )≈45–60 m s −1 (justified by the high electric field ≈3 × 10 7 V m −1 , see Wilamowski et al . [42] and Nestoklon et al . [43] ). The fit then extracts a dipole size r ≈1–2 nm for both values of E VS . The good agreement between the calculations and the experiment, as well as the presence of a hot-spot at the point of degeneracy between Zeeman and VS, provide strong evidence of our ansatz that the spin relaxation is predominantly due to a new mechanism: that of mixing with the excited valley states via Rashba/Dresselhaus-like SOC in the presence of interface disorder. Both the splitting at the anticrossing, equation (4), and the inter-valley relaxation, equation (6), depend crucially on the size of the dipole matrix element, r , predicting a fast phonon relaxation of ≈10 7 –10 8 s −1 for r =1–3 nm, at the hot-spot of Fig. 2d . This confirms our core findings that when spin-valley states anticross, the inter-valley rates are fast for these samples, with the only available relaxation mechanism being the inter-valley decay. We point out that these relaxation rates are expected to be sample/material-dependent, given the effect of interface disorder on valley mixing. We now examine the case where N =2 electrons, and investigate the dependence of the relaxation rate on the magnetic field at a fixed VS ( E VS =0.58 meV). We note that the energy levels accessible for loading the second electron in the dot, when the N =1 spin-down ground state is already occupied, are either the singlet ( S ) or the two lower triplets ( T − , T 0 ), whereas the higher triplet ( T + ) would require a spin flip and is, therefore, not readily accessible (see Fig. 3a ). In general, for triplet states, the antisymmetry of the two-electron wavefunction requires one electron to occupy a higher energy state. For our multi-valley QD ( Fig. 1f ), this requirement is fulfilled when the two electrons occupy different valley states (see Fig. 3a ). For low fields, the ground state is S and the triplets have higher energies. This results in excited states (triplets) that extend over two valleys and relax to a single-valley ground state (singlet). 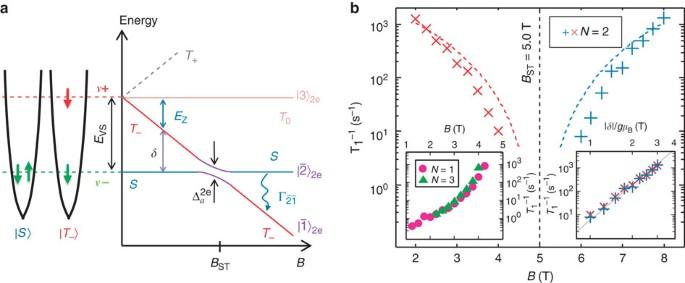Figure 3: Spin-valley relaxation for multi-electron occupancy. (a) Energy diagrams of the two-electron spin-valley states in the dot’s potential well (left) and as a function ofBfield (right). Dashed line indicates thatT+is not accessible (see text). (b) Relaxation rate as a function ofBfield forN=2 andEVS=0.58 meV. Red (blue) crosses represent data points at fields smaller (larger) than the anticrossing point. Dashed lines are the calculated rates fitted withr2e=4.76 nm. Right inset: Data from the main graph re-plotted as a function of the modulus of the detuning energy,δ. Points of equal absolute detuning have nearly the same decay rates.δ5dependence (grey line) is a guide for the eye. Left inset: Relaxation rate as a function ofBfield forN=3 andEVS=0.58 meV. Results forN=1 are also shown for comparison. Figure 3: Spin-valley relaxation for multi-electron occupancy. ( a ) Energy diagrams of the two-electron spin-valley states in the dot’s potential well (left) and as a function of B field (right). Dashed line indicates that T + is not accessible (see text). ( b ) Relaxation rate as a function of B field for N =2 and E VS =0.58 meV. Red (blue) crosses represent data points at fields smaller (larger) than the anticrossing point. Dashed lines are the calculated rates fitted with r 2e =4.76 nm. Right inset: Data from the main graph re-plotted as a function of the modulus of the detuning energy, δ . Points of equal absolute detuning have nearly the same decay rates. δ 5 dependence (grey line) is a guide for the eye. Left inset: Relaxation rate as a function of B field for N =3 and E VS =0.58 meV. Results for N =1 are also shown for comparison. Full size image As the magnetic field is increased, S and T − undergo an avoided crossing ( B ≡ B ST ), and then T − becomes the ground state. We adjust the levels of our pulsed read-out protocol so that during the load phase only S and T − are below the reservoir’s Fermi energy, whereas, during the read phase, the Fermi energy is positioned within the singlet–triplet (ST) energy gap. As a consequence, for B < B ST ( B > B ST ) a T − ( S ) state would be signalled with a current transient, and relaxation rates can be extracted as for the N =1 occupancy. The experimental relaxation rates in Fig. 3b show a strongly non-monotonic behaviour, approaching an absolute minimum at the anticrossing point ( B ST =5 T). The trend is strikingly symmetric, as can be appreciated when is plotted against the detuning energy, as shown in the right inset. This symmetry is reflected in the QD energy spectrum ( Fig. 3a ), as far as the detuning δ is concerned. For B < B ST , the ST energy gap decreases with increasing B , resulting in slower relaxation rates. By contrast, for B > B ST , the ST energy gap increases with increasing field, and so does the relaxation rate. As opposed to the one-electron case, we note that the two-electron eigenstates anticrossing leads to a minimum in the relaxation rate (cold-spot), defined by a splitting at the anticrossing, , of the same order as that of equation (4) (see Fig. 3a and Supplementary Note 3 ). The occurrence of this minimum does not strictly depend on the nature of the states involved in the decay (spin-like, valley-like, orbital-like or admixtures). It is due to the fact that the avoided crossing takes place between the ground and the first excited state, whereas for the case N =1 it involves the first and the second excited states without affecting the ground state. To model the two-electron case, we build the wavefunctions for S and T − from the single-particle states by considering the Coulomb interaction as a perturbing averaged field. The corresponding states are defined as , . Next, the additional perturbation given by SOC leads to renormalized eigenstates that are admixtures of singlet and triplet: being similar forms to equations (2) and (3). As we show in Supplementary Note 3 , by evaluating the electron–phonon Hamiltonian matrix element for the transition between these states, one finds that it coincides in its form with its one-electron counterpart for . Therefore, we can conclude that the corresponding relaxation rate, , has the same functional form as those derived in equation (8), although the matrix elements for the two cases will be different (see Supplementary Note 3 ). The dashed lines in Fig. 3b represent the calculated rates that are fitted to the experimental data similarly to the case where N =1. Once again, the model convincingly reproduces the main features of the experimental trend, in particular the rates for fields away from the anticrossing, together with the symmetry of the characteristics with respect to B ST . Further work may be needed to improve the fit in the vicinity of the anticrossing point. We also measured the relaxation rates for N =3 electrons. When the QD occupancy is set at N =2, the lower valley is fully occupied and for low B fields the ground state is a singlet. In this condition, the read-out protocol is adjusted to probe spin relaxation within the upper valley upon loading/unloading of the third electron. By keeping E VS =0.58 meV and using the same methodology described before, we measure relaxation rates for the third electron spin state. We find that there is no significant difference between the spin relaxation rates for N =3 and N =1, as shown in the left inset of Fig. 3b . Two main conclusions can be drawn from this. First, we can infer that the effect of electron–electron interactions on the multi-valley spectrum may be negligible [44] , which is plausible. Indeed, for valley three-electron states, two electrons are just ‘spectators’, so that the remaining electron establishes the same energy level structure as in Fig. 2c , and the Coulomb corrections do not affect the VS. Second, as we report in Yang et al . [41] , in small QDs for higher occupancies a significantly reduced energy separation between the ground state and the first excited orbital state is observed. This would introduce a non-negligible perturbation on the relaxation if this were affected by the orbital degree of freedom. Hence, the similarities in behaviour in terms of decay rates are a further indication that for our QD the dominant relaxation mechanism resides in the degree of spin-valley admixing, as opposed to the spin–orbit admixing relevant for other semiconductor systems [28] . Valley splitting control We now turn to the experimental demonstration of accurate control of the VS, E VS , via electrostatic gating. To determine E VS , we use two different experimental approaches. One utilizes the rapid increase in spin relaxation at the hot-spot, and is applicable in the low-magnetic-field regime. The other is based on magnetospectroscopy, and is relevant for high fields. The first technique stems from the fact that the hot-spot can be reliably detected by monitoring the spin-up probability as a function of magnetic field. In Fig. 4a , we show measurements of the spin-up probability performed with the same method as the one used to evaluate spin lifetimes (see Supplementary Note 2 ). We see that the probability of detecting a spin-up electron decreases significantly at some magnetic fields. A sudden drop of the spin-up fraction in a narrow range of field identifies the increase in relaxation rate associated with the hot-spot. Given that valley and Zeeman splittings coincide at the hot-spot, one can extract the valley separation as E VS = gμ B B HS , where B HS is defined as the field at which the hot-spot is observed. For varying gate-voltage configurations, we scan B in the range 2.8 T< B <5 T, and identify B HS by setting an arbitrary probability threshold (green-shaded area in Fig. 4a ) below which the hot-spot is assumed to occur. The use of this technique is limited to B <5 T because the lifetime drop at the hot-spot can be therein confidently assessed. At higher fields the relaxation becomes increasingly fast and its enhancement at the hot-spot is indistinguishable within our measurement bandwidth (≈10 kHz). 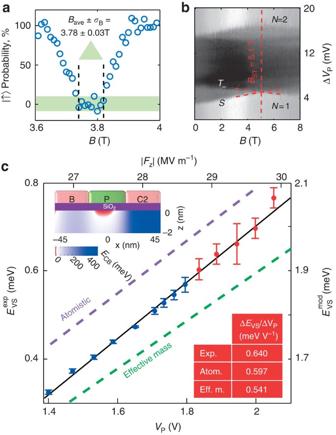Figure 4: Tunability of the VS via gate-voltage control. (a) Spin-up probability as a function of magnetic field forVP=1.59 V. The occurrence of a hot-spot minimizes the spin-up fraction and allows one to extractBHS(shaded area) and, in turn,EVS. (b) Pulsed-voltage magnetospectroscopy showing dISET/dVPatN=1→2 transition. A square pulse of amplitude 16 mV at 287 Hz is applied to gate P. The evolution of the energy difference between the singlet state (light grey) and the triplet state (dark grey) allows one to extractBST(dashed line) and, in turn,EVS. (c) Valley splitting as a function of plunger gate voltage (bottom axis) and modulus of interface vertical electric field in the QD (top axis). Blue and red dots show the valley separation (left axis) measured with hot-spot and magneto-spectroscopic techniques, respectively. Error bars indicate standard deviations for the measured values. The linear fit (solid line) indicates a valley tunability of 0.640 meV V−1. Dashed lines are calculations performed via atomistic (purple) and effective mass (green) methods (right axis). Bottom inset: Table comparing calculated and experimental tunabilities. Top inset: TCAD simulation of the conduction band profile atVP=1.4 V in the (x,z) plane. Negative energy region in red reveals where the dot is formed. Figure 4: Tunability of the VS via gate-voltage control. ( a ) Spin-up probability as a function of magnetic field for V P =1.59 V. The occurrence of a hot-spot minimizes the spin-up fraction and allows one to extract B HS (shaded area) and, in turn, E VS . ( b ) Pulsed-voltage magnetospectroscopy showing d I SET /d V P at N =1→2 transition. A square pulse of amplitude 16 mV at 287 Hz is applied to gate P. The evolution of the energy difference between the singlet state (light grey) and the triplet state (dark grey) allows one to extract B ST (dashed line) and, in turn, E VS . ( c ) Valley splitting as a function of plunger gate voltage (bottom axis) and modulus of interface vertical electric field in the QD (top axis). Blue and red dots show the valley separation (left axis) measured with hot-spot and magneto-spectroscopic techniques, respectively. Error bars indicate standard deviations for the measured values. The linear fit (solid line) indicates a valley tunability of 0.640 meV V −1 . Dashed lines are calculations performed via atomistic (purple) and effective mass (green) methods (right axis). Bottom inset: Table comparing calculated and experimental tunabilities. Top inset: TCAD simulation of the conduction band profile at V P =1.4 V in the ( x , z ) plane. Negative energy region in red reveals where the dot is formed. Full size image In order to evaluate E VS at higher magnetic fields, we use a more conventional magneto-spectroscopic approach, as shown in Fig. 4b . By employing the same gate-pulsed technique used for the charge stability experiments (see Supplementary Note 1 ), we focus on the singlet–triplet ground-state transition as we load the second electron into the dot (that is, N =1→2 transition) in the range 5 T< B <6.5 T. This is clearly identified as the point where the S (light grey feature) and T − (dark grey feature) states cross. Here, E VS = gμ B B ST , as seen in Fig. 3a . The data points in Fig. 4c represent the measured valley separation as a function of V P , obtained by means of the aforementioned techniques. The solid line fit shows remarkable consistency between the two sets of data and reveals that E VS depends linearly on the gate voltage over a range of nearly 500 μeV, with a slope of 640 μeV V −1 . In order to keep constant the dot’s occupancy and tunnelling rates for different V P , a voltage compensation is carried out by tuning gates C1 and B accordingly. We note that we previously reported VSs of comparable magnitude (few hundreds of μeV) in devices realized with the same technology [41] , [45] . However, to our knowledge, this is the first demonstration of the ability to accurately tune the VS electrostatically in a silicon device. A linear dependence of the VS with respect to the vertical electric field has been predicted for 2DEG systems via effective mass theory [7] , [9] , [10] . A similar dependence for MOS-based QDs [46] has also been reported by employing atomistic tight-binding calculations [47] . In order to compare our experimental finding with the theoretical predictions, we simulate the vertical electric field ( F Z ) in the vicinity of the dot for the range of gate voltages used in the experiments. We employ the commercial semiconductor software ISE-TCAD [48] to model the device’s electrostatic potential, and thereby the electric fields in the nanostructure. For this purpose, TCAD solves the Poisson equation with an approximation of Newton’s iterative method [49] to obtain convergence at low temperatures. The spatial extent of the dot is identified by regions where the calculated conduction band energy drops below the Fermi level (red area in the top inset of Fig. 4c ). Note that our calculations are performed on a three-dimensional geometry identical to the real device with the only free parameter being the amount of offset interface charge. This is adjusted to match the experimental threshold voltage of the device ( V th =0.625 V), as explained in the Supplementary Note 4 . The computed variation of interface electric field with gate voltage V P is used to determine the VS according to both the atomistic [46] and effective mass [7] predictions. Dashed lines in Fig. 4c depict the trends for both approaches, with both exceeding by more than 1 meV of the measured values. Despite this offset, the atomistic calculations give a tunability of the VS with gate voltage, Δ E VS /Δ V P , in good agreement with the experiments. The calculated value of 597 μeV V −1 agrees with the measured value to within less than 7%. The value of 541 μeVV −1 calculated using the effective mass approach reveals a larger deviation (≈15%) from the experiments. The presence of an offset in the computed VS may be due to the contribution of surface roughness that is not accounted for in the models, and is thought to be responsible for a global reduction of E VS [8] , [10] , [11] , [12] , [50] , [51] . We emphasize, however, that the gate tunability would remain robust against this effect, which is not dependent on electric field. In this work, we have shown that the VS in a silicon device can be electrostatically controlled by simple tuning of the gate bias. We used this VS control, together with spin relaxation measurements, to explore the interplay between spin and valley levels in a few-electron quantum dot. The relaxation rates for a one-electron system exhibit a dramatic hot-spot enhancement when the spin Zeeman energy equals the VS, whereas for a two-electron system the rates reach a minimum at this condition. We found that the known mechanisms for spin relaxation, such as the admixing of spin and p orbital states, were unable to explain the key features of the experimental lifetime data, and so introduced a novel approach based on admixing of valley and spin eigenstates. Our theory, which showed good agreement with experiment, implies that spin relaxation via phonon emission due to spin-orbit coupling can occur in realistic quantum dot systems, most likely due to interface disorder. Our results show that by electrical tuning of the VS in silicon quantum dots, it is possible to ensure the long lifetimes ( T 1 >1 s) required for robust spin qubit operation. Despite this, the excited valley state will generally be lower than orbital states in small quantum dots, placing an ultimate limit on the lifetimes accessible in very small dots, due to the spin-valley mixing described above. Electrical manipulation of the valley states is also a fundamental requirement to perform coherent valley operations. However, the experimental relaxation rate at the observed hot-spot was found to be fast ( >1 kHz) for our devices, implying a fast inter-valley relaxation rate. Finally, in the context of realizing scalable quantum computers, these results allow us to address questions of device uniformity and reproducibility with greater optimism. Indeed, our work suggests that issues related to the wide variability of the VS observed in silicon nanostructures to date can shift from the elusive atomic level (surface roughness, strain, interface disorder) to the more accessible device level, where gate geometry and electrostatic confinement can be engineered to ensure robust qubit systems. Device fabrication The samples fabricated for these experiments are silicon MOS planar structures. The high purity, near intrinsic, natural isotope silicon substrate has n+ ohmic regions for source/drain contacts defined via phosphorous diffusion. High quality SiO 2 gate oxide is 8 nm thick and is grown by dry oxidation at 800 °C. The gates are defined by electron-beam lithography, Al thermal evaporation and oxidation. Three layers of Al/Al 2 O 3 are stacked and used to selectively form a 2DEG at the Si/SiO 2 interface and provide quantum confinement in all the three dimensions. Measurement system Measurements are carried out in a dilution refrigerator with a base temperature T b ≈40 mK. Flexible coaxial lines fitted with low-temperature low-pass filters connect the device with the room-temperature electronics. In order to reduce pick-up noise, the gates are biased via battery-powered and opto-isolated voltage sources. The SET current is amplified by a room-temperature transimpedance amplifier and measured via a fast-digitizing oscilloscope and a lock-in amplifier for the single-shot and energy spectrum experiments, respectively. Gate voltage pulses are produced by an arbitrary wave-function generator and combined with a DC offset via a room-temperature bias-tee. How to cite this article: Yang, C. H. et al . Spin-valley lifetimes in a silicon quantum dot with tunable valley splitting. Nat. Commun. 4:2069 doi: 10.1038/ncomms3069 (2013).